Stationary domain wall contribution to enhanced ferroelectric susceptibility In ferroelectrics, the effect of domain wall motion on properties has been widely studied, but non-motional or stationary contributions from the volume of material within the domain wall itself has received less attention. Here we report the measurement of stationary domain wall contributions to permittivity in PbZr 0.2 Ti 0.8 O 3 films. Studies of (001)-, (101)- and (111)-oriented epitaxial films reveal that (111)-oriented films, in which the motional domain wall contributions are frozen out, exhibit permittivity values approximately three times larger than the intrinsic response alone. This discrepancy can only be accounted for by considering a stationary contribution from the domain wall volume of the material that is 6–78 times larger than the bulk response, and is consistent with predictions of the enhancement of susceptibilities within 90° domain walls. This work offers new insights into the microscopic origin of dielectric enhancement and provides a pathway to engineer the dielectric response of materials. The search for ferroelectric materials with high electric field (dielectric), stress (piezoelectric) and thermal (pyroelectric) susceptibilities has garnered much attention in recent years, as these materials serve as the foundation for modern memory [1] , [2] , [3] , sensor and actuator [4] , [5] , [6] , and thermal imaging and infrared detector systems [7] , [8] , [9] . To ultimately understand the nature of such responses, it is imperative to understand the various contributions to the susceptibility in these complex materials. Since ferroelectrics typically possess complex domain structures with homogeneously polarized domains separated by domain walls, the susceptibility consists of two major contributions. The first is the so-called intrinsic contribution arising from the change in the polarization to an applied stimulus within the bulk of the domains. The second is the so-called extrinsic contribution, which refers to the contribution that arises due to the motion of domain walls under an applied stimulus [10] , [11] , [12] , [13] , [14] , [15] , [16] , [17] , [18] . Beyond the motional extrinsic contribution from domain walls, various reports have highlighted the potential importance of what has been alternatively called a stationary or frozen contribution that arises from the response of the volume of the ferroelectric material within the finite width of the domain walls to an applied stimulus irrespective of any lateral displacements or deformations of the wall [19] , [20] , [21] , [22] . As early as 1970s, the importance of these various contributions to ferroelectric susceptibility was already under investigation. Early studies of dielectric permittivity in BaTiO 3 revealed what was suspected to be a large domain wall contribution to permittivity even at excitation fields where the lateral displacement of domain walls was unlikely [23] . Subsequent theoretical studies probed the possibility of the weak measurement fields inducing nuclei on the existing domain walls and thus promoting protuberance-type oscillation, but revealed that these could only account for a small fraction of the observed permittivity change [24] . Soon after this it was conjectured that the material within the domain walls themselves could possess significantly enhanced dielectric permittivity [19] , [25] . Such models suggested that 180° domain walls in BaTiO 3 could possess permittivity almost an order of magnitude larger than the bulk of the domains. More recently, advanced Ginzburg–Landau–Devonshire (GLD) models have probed the role of polarization gradients near 90° domain walls in BaTiO 3 to suggest that such domain walls could give rise to an enhancement of susceptibilities between 1.1 and 1,000 times larger than the bulk [22] . Despite these predictions as to the potential importance of such stationary contributions, it has proven difficult to quantitatively measure and isolate the stationary contribution (possibly because of the small relative volume associated with domain walls in most samples). In turn, much work on polydomain ferroelectrics has neglected the stationary contribution and focused solely on enhancements that can be explained by motional extrinsic contributions. Regardless, it is clear that in order to fully understand the response of a ferroelectric to an applied stimulus, one must consider not only the response of the bulk material within the domains but also the response of the domain walls to the applied stimuli. Here we use a combination of theoretical and experimental approaches to investigate the effect of 90° domain walls on the dielectric permittivity of (001)-, (101)- and (111)-oriented PbZr 0.2 Ti 0.8 O 3 thin films. Using phenomenological GLD models we calculate the intrinsic and motional extrinsic contributions to permittivity for these different film orientations. Thin-film epitaxy is employed to synthesize highly controlled model versions of these films. The choice of these three orientations enables us to tune the density of domain walls and thus the relative magnitude of the stationary domain wall contribution to permittivity. In particular, we observe that in (111)-oriented films we can produce high-density, nanotwinned domain structures made entirely of 90° domain walls. Subsequent comparison of the measured dielectric permittivity and the GLD models reveals a large enhancement of the permittivity that is consistent with a large stationary domain wall contribution. From these measurements we find that the magnitude of the stationary domain wall response is 6–78 times larger than the intrinsic response within a domain. These observations provide the first quantitative measurement of the stationary contribution of domain walls and reveal that the large responses at the domain wall can be utilized to improve the overall dielectric susceptibilities. GLD models In order to study the intrinsic and motional extrinsic contributions to the dielectric permittivity, we considered thin films of the tetragonal ferroelectric PbZr 0.2 Ti 0.8 O 3 grown epitaxially on (001)-, (101)- and (111)-oriented cubic substrates. We utilize the Helmholtz free energy formalism applicable to ferroelectric films with dense domain structures to calculate the domain structures and dielectric susceptibilities as a function of substrate orientation and epitaxial strain [26] , [27] , [28] . Consistent with prior approaches, we assume homogeneous strain fields within the domains and neglect the domain wall self-energies and inter-domain electrostatic interactions. Applying short-circuit electrical boundary conditions, the free energy of the system is minimized as a function of the in-plane strain imposed by the substrate so that we can calculate the equilibrium polarizations ( P 1 , P 2 , P 3 ) and domain fractions. Using these models, we can then calculate explicitly the out-of-plane permittivity ( ) as the sum of the intrinsic (the first term) and the motional extrinsic (the second term) contributions [17] , [26] , [27] , [28] , [29] as where is the fraction of domains with polarization P i , F is the free energy formalism, is the out-of-plane polarization component of P i and E is the electric field along the substrate normal (for details see Supplementary Note 1 ). Note that these models exclude stationary domain wall contributions from the portion of the material contained within the finite width of the domain walls. The domain volume fraction ( ) and dielectric permittivity ( ) have been calculated numerically for all three orientation variants as a function of misfit strain ( Fig. 1 ). For comparison, the strain regime that was explored was chosen to correspond to theoretically predicted epitaxial strains that give rise to c/a/c/a polydomain structures in (001)-oriented films [26] , [30] . Schematic illustrations of the expected domain structures in each film orientation are provided (see Supplementary Fig. 1 ). In (001)-oriented films, the volume fraction of c domains ( ) is observed to decrease with increasing tensile strain, while the volume fraction of a domains ( and ) increases as a result of the tensile strain that favors in-plane oriented polarization ( Fig. 1a ). A similar competitive trend is observed in (101)-oriented films where the population of the in-plane polarized domains ( ) increases and the fraction of out-of-plane polarized domains ( and ) deceases with increasing strain ( Fig. 1b ). This is not the case for the (111)-oriented films, however, which due to symmetry, possess three energetically degenerate domain types and thus an equal volume fraction ( ) of each domain separated by 90° domain walls at all values of misfit strain considered ( Fig. 1c ). Correspondingly, we can observe the impact of changing film orientation on ( Fig. 1d–f ). In general, the intrinsic contribution to permittivity increases as the substrate normal is inclined more towards the [100], which is similar to the monodomain case where the permittivity exhibits higher values along non-polar directions (that is, [111]) than polar directions (that is, [001]) in tetragonal ferroelectrics [31] , [32] . This is due to the anisotropic dielectric response of PbZr 0.2 Ti 0.8 O 3 where the permittivity along the [100] is larger than that along the [001] [32] . Thus the enhanced intrinsic response in (101)- and (111)-oriented films arises from the fact that additional intrinsic contributions are activated. It is also noted that the increasing tensile strain results in an increasing intrinsic response in the (001)-oriented films, which behaves in an opposite trend as compared to the (101)- and (111)-oriented films due to the fact that the intrinsic response of each polarization variant in (001)-oriented films increases while this component in (101)- and (111)-oriented films decreases with increasing tensile strain. At the same time, the relative contribution from the motional extrinsic response decreases as we move from (001)- to (101)-oriented films (as a result of less preferential alignment of the electric field with a single polarization variant) and completely vanishes in (111)-oriented films owing to the constant volume fraction of the three polarization variants, which is independent of the electric field. Similar to BaTiO 3 single crystals poled along [111] (ref. 33 , 34 ), the extrinsic contribution from domain wall motion will be ‘frozen out’ in (111)-oriented PbZr 0.2 Ti 0.8 O 3 films. In addition, the motional extrinsic contribution for (001)- and (101)-oriented films behaves differently with increasing strain, leading to an increasing and decreasing extrinsic contribution in (001)- and (101)-oriented films, respectively. Despite these differences, across the entire strain regime studied here and for all three film orientations, the overall predicted is found to exist in a rather narrow range between 220 and 290. 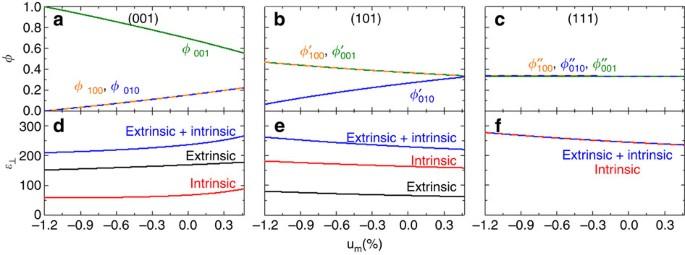Figure 1: Domain and permittivity evolution in PbZr0.2Ti0.8O3thin films. Using Ginzburg–Landau–Devonshire models, the volume fraction of polarization variants () and out-of-plane, room temperature dielectric permittivity () are predicted as a function of mismatch strain (um). The evolution of ? is provided for (a) (001)-, (b) (101)- and (c) (111)-oriented films including the relative fraction of different polarization variants (referenced to the cardinal directions of the lattice, [100], [010] and [001]). The evolution of the intrinsic (red), extrinsic (black), and total (blue)is provided for (d) (001)-, (e) (101)-, and (f) (111)-oriented films. Figure 1: Domain and permittivity evolution in PbZr 0.2 Ti 0.8 O 3 thin films. Using Ginzburg–Landau–Devonshire models, the volume fraction of polarization variants ( ) and out-of-plane, room temperature dielectric permittivity ( ) are predicted as a function of mismatch strain (u m ). The evolution of ? is provided for ( a ) (001)-, ( b ) (101)- and ( c ) (111)-oriented films including the relative fraction of different polarization variants (referenced to the cardinal directions of the lattice, [100], [010] and [001]). The evolution of the intrinsic (red), extrinsic (black), and total (blue) is provided for ( d ) (001)-, ( e ) (101)-, and ( f ) (111)-oriented films. Full size image Thin film growth and domain structures We proceed to examine model ferroelectric thin films of different orientations experimentally. We focus on 150 nm PbZr 0.2 Ti 0.8 O 3 /10 nm SrRuO 3 or La 0.7 Sr 0.3 MnO 3 /SrTiO 3 (001), (110) and (111) heterostructures grown via pulsed-laser deposition (see Methods for details). The domain structure of the films was probed via piezoresponse force microscopy (PFM). In (001)-oriented PbZr 0.2 Ti 0.8 O 3 thin films, we observe c/a/c/a domain structures that are commonly seen in tetragonal ferroelectric thin films and consist of majority out-of-plane polarized c and in-plane polarized a domains separated by 90° domain walls ( Fig. 2a ) [35] , [36] . The density of 90° domain walls is known to increase with increasing tensile strain, which corresponds to an enhancement of the motional extrinsic contribution to the low-field permittivity in (001)-oriented films [17] , [26] , [27] . Considerably, less work in this vein, however, has been undertaken for (101)- and (111)-oriented films [37] . 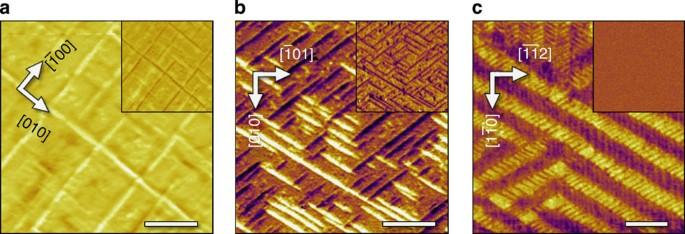Figure 2: Domain structure characterization of PbZr0.2Ti0.8O3films. Piezoresponse force microscopy images showing lateral (mixed phase (θ) and amplitude (A),Acosθ) and vertical (mixed phase (θ) and amplitude (A),Acosθ, inset) contrast for equilibrium domain structures of (a) (001)-, (b) (101)- and (c) (111)-oriented PbZr0.2Ti0.8O3thin films. Scale bar: 500 nm. Figure 2: Domain structure characterization of PbZr 0.2 Ti 0.8 O 3 films. Piezoresponse force microscopy images showing lateral (mixed phase ( θ ) and amplitude ( A ), A cos θ ) and vertical (mixed phase ( θ ) and amplitude ( A ), A cos θ , inset) contrast for equilibrium domain structures of ( a ) (001)-, ( b ) (101)- and ( c ) (111)-oriented PbZr 0.2 Ti 0.8 O 3 thin films. Scale bar: 500 nm. Full size image Thus, here we provide detailed studies of domain structures and permittivity in (101)- and (111)-oriented films. In the (101)-oriented films the PFM images reveal a mixed domain pattern where the majority of the sample is made up of domains with polarization along the [001], which is oriented at an angle of ~43.6° from the plane of the film, while the remaining structure consists of stripe-like domains possessing only in-plane polarization components pointing along the [010] or ( Fig. 2b ). In (111)-oriented films, however, a complex metastable domain structure was observed in the as-grown state (see Supplementary Fig. 2 ), and in order to probe the equilibrium domain structure, the samples were poled with a series of +/−6 V biases applied locally to a PFM tip to switch a 2.5 μm × 2.5 μm region (samples were switched between 2 and 6 times). Following such poling, a complex, ordered, nanotwinned domain pattern with a high density of uncharged 90° domain walls was observed ( Fig. 2c ). The observed domain structure is the result of the tiling of three types of domain bands, separated by 120° with average domain band widths of ~300 nm. Within each domain band, the domain structure consists of a mixture of all three degenerate polarization variants (pointing along the , and , which are oriented at an equal angle of ~33.9° from the plane of the film) distributed into two sub-bands, with each sub-band being made-up of only two of the polarization variants, consistent with prior predictions [38] . Reciprocal space-mapping studies confirm the above polydomain structures for the various film orientations (see Supplementary Fig. 3 ). Regardless of the film orientation, the PFM studies indicate the presence of no 180° domain walls as a result of the preferential out-of-plane direction of the polarization that is induced by the asymmetric electrical boundary conditions (that is, the presence of a bottom electrode). Thus, in comparison to traditional bulk ceramic samples, these films provide a well-characterized model system exhibiting controllable domain structures possessing only a single type of domain wall (that is, 90°). The PFM analysis further allows for the direct quantification of the domain structures—in particular, the determination of the domain wall density (λ, defined as the total length of domain walls in a given area) and the volume fraction of minority domains ( , defined as the volume fraction of the domain type that possesses the smallest population among all polarization variants in the case of a poled film). Further definition and schematic illustrations of these minority domains are provided (see Supplementary Fig. 1 ). In (001)- and (101)-oriented films, the minority domain represents the domain with the polarization pointing in the plane-of-the-film (along the [100], [010] and [010], [0 0], respectively). Due to symmetry in (111)-oriented films, however, one can select any of the three polarization variants as the minority domain as they all form an equal angle with the normal direction of the substrate and occur in equal fractions. Details of the analysis are provided in the Supplementary Information (see Supplementary Fig. 4 and Supplementary Note 2 ), but briefly, image analysis of the PFM domain structure images allows for the selection and measurement of the perimeter and area of all domain types, and hence the direct measurement of λ and the area fraction of the domains. To estimate , we have assumed a uniform width of the domains throughout the thickness of the film [39] , [40] , [41] , [42] . It should be noted that this assumption matches the assumptions of the GLD models (or, in other words, matches the ideal domain structure that would be predicted from such models), but might slightly overestimate the volume density if the domains are more wedge-shaped [43] . Regardless, this potential slight discrepancy has little to no impact on the overall conclusion of the data below. The values of λ and are provided ( Table 1 ). From this analysis, it is clear that the (111)-oriented films possess domain wall densities that are at least 3–5.5 times larger than the values for (001)- and (101)-oriented films, and that the experimentally observed value is consistent with the degeneracy of the three polarization variants in (111)-oriented films calculated from the GLD models. Table 1 Domain structure analysis of PbZr 0.2 Ti 0.8 O 3 films. Full size table This work reveals that in addition to the use of epitaxial strain [44] , film thickness [36] and film composition [45] to manipulate domain structures in ferroelectrics, film orientation is another effective route by which to control the domain structure and domain wall density. In fact, (111)-oriented films enable the study of domain structures and densities that are not possible in other orientations at these film thicknesses. This enhanced density of domain walls will boost the contribution of such features to the overall response to applied stimuli. Furthermore, due to the degeneracy of the different domain variants, the extrinsic contribution from the domain walls is expected to be solely due to the stationary domain wall contributions (not motional extrinsic contributions), which presents a unique opportunity to study the stationary response of domain walls to external stimuli quantitatively. Dielectric properties of the films Detailed dielectric characterization of symmetric capacitor structures of the various orientations of films was performed (see Methods for details). For all measurements reported herein, the capacitor structures were subjected to current–voltage and ferroelectric characterization first, including multiple switching processes to assess the nature of the hysteresis loops and to assure measurements of poled capacitors only. Only capacitors showing symmetric current–voltage response and well-saturated, symmetric and imprint-free hysteresis loops across the frequency range 1 Hz–10 kHz were probed (see Supplementary Figs 5,6 and Supplementary Note 3 ). The quality of the films and the accuracy of the measurements of domain wall density and domain fraction are confirmed using the procedure of ref. 46 , and the estimated values of polarization along the [001] are found to be approximately constant across the different orientations. Subsequently, the room temperature low-field dielectric permittivity ( ) was measured with an AC excitation field with an amplitude of 50 mV (in the frequency range from 0.1 to 10 kHz). The amplitude of the applied field was confirmed to be in the reversible regime via Rayleigh studies (see Supplementary Fig. 7 and Supplementary Note 3 ). The (001)- and (101)-oriented films show values within the range =185–267, while the (111)-oriented films exhibit significantly enhanced =654–691 across this same frequency range ( Fig. 3 ). 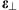Figure 3: Frequency dependence of permittivity () in PbZr0.2Ti0.8O3thin films. The solid symbol lines showmeasured at an AC excitation of 50 mV for (001)-, (101)- and (111)-oriented PbZr0.2Ti0.8O3thin films. The error bars show the standard deviation from the measurement of eight different capacitors on a given sample. The dashed lines show the predicted(including intrinsic and extrinsic contributions) from the Ginzburg–Landau–Devonshire models. Figure 3: Frequency dependence of permittivity ( ) in PbZr 0.2 Ti 0.8 O 3 thin films. The solid symbol lines show measured at an AC excitation of 50 mV for (001)-, (101)- and (111)-oriented PbZr 0.2 Ti 0.8 O 3 thin films. The error bars show the standard deviation from the measurement of eight different capacitors on a given sample. The dashed lines show the predicted (including intrinsic and extrinsic contributions) from the Ginzburg–Landau–Devonshire models. Full size image A comparison of these measured values with the calculated permittivity from the GLD models was made by extracting the data point from Fig. 1 at the experimentally measured given in Table 1 . The calculated (including both intrinsic and extrinsic contributions) for all three orientations shows small differences (all orientations are predicted to have values between 220 and 250), which agrees well with the experimental results for (001)- and (101)-oriented films. The (111)-oriented films, however, show a significant discrepancy between the experimentally measured and theoretically predicted values. As is noted in the discussion of the GLD model for the (111)-oriented films, all three degenerate polarization variants are present in equal volume fractions, and these fractions will not vary with the application of an electric field, thus leading to an absence of a motional extrinsic contribution. The experimental results, however, imply that for (111)-oriented films is greatly enhanced with increasing domain wall density (or decreasing average domain width). This enhancement suggests that the high density of domain walls in the (111)-oriented films could potentially give rise to a stationary domain wall contribution that can enhance the permittivity. To further quantify this stationary domain wall contribution, we utilized an equivalent electrical circuit model to calculate the effective domain wall permittivity. Previous studies [38] suggest that the 90° domain walls present in the (111)-oriented heterostructures, by symmetry and to avoid charged domain boundaries, should be inclined from the plane of the film at an angle of ~33.9°. When applying electric field along the normal direction of the film, the electric field lines should proceed straight along the normal direction within the domains, but will be deflected from the vertical direction within the domain walls according to the appropriate Maxwell equation (see Supplementary Fig. 8 ). Thus an appropriate model of an equivalent circuit for this system requires that we treat the domain and domain walls as capacitors in series where the effective thickness of each capacitor is geometrically calculated based on the path length of the field within that element. Detailed description of the calculation process has been provided in Supplementary Note 4 . Using the experimentally measured average domain width (~40 nm), the experimentally measured (~670), the calculated intrinsic dielectric permittivity (~245) and by assuming the domain wall width to be (conservatively) 1–10 nm [39] , [40] , [41] , [42] , [47] , one can estimate to be 1,500–19,000, which is 6–78 times larger than the expected intrinsic response within a domain. As noted above, recent theoretical work using a decoupling approximation and GLD modelling suggests the possibility of up to a thousandfold enhancement of the dielectric susceptibility and piezoelectric response across 90° domains walls in tetragonal ferroelectrics (like those found in our samples) due to structural and polarization inhomogeneities within the domain wall region [22] . Our work, in turn, experimentally demonstrates that high-density, stationary 90° domain walls could provide significantly enhanced dielectric response in the epitaxial thin films, particularly at large domain wall densities. The above results show that the application of electric field along certain non-polar directions in tetragonal ferroelectrics can be used to effectively ‘freeze out’ the domain wall motion, and thus enables us to probe the stationary domain wall contribution to susceptibility. This is aided by the fact that growth of (111)-oriented films produces a configuration of numerous degenerate polarization variants, enables the application of electric fields along non-polar directions and produces domain wall densities high enough to promote the stationary domain wall contribution to be comparable in magnitude to the intrinsic response from the bulk of the domains. These observations, made possible by the simplicity of the engineered domain structure in the epitaxial thin films, and our ability to directly probe the type, density and response of these domain wall structures in different orientations produce a complementary approach to the study of ferroelectric single crystals with fields applied along different crystallographic directions and provide an opportunity to re-examine the importance of domain structure in controlling field-induced response. These studies suggest that the stationary domain wall contribution to ferroelectric susceptibility should be given additional attention for its potential to enhance overall material performance. To date, the understanding of intrinsic and motional extrinsic responses in these materials has led researchers to decrease the average domain size to enhance susceptibilities. The observed increase in performance, although likely partially enhanced by extra-motional extrinsic contributions, could also be strengthened by simultaneous turn-on of stationary domain wall contributions. In one extreme case one could imagine that in systems controlled to have extremely fine domain structures, domain wall–domain wall interactions could lessen the extent of motional extrinsic contributions while still exhibiting enhancements in susceptibility from the stationary domain wall contribution. The failure to consider such stationary domain wall contributions, in turn, could result in the attribution of performance enhancements to the wrong feature in the material. Our work suggests that motional extrinsic contributions to permittivity are (at best) a factor of two times larger than the intrinsic response, while stationary domain wall contributions could be as large as 6–78 times larger than the intrinsic response [48] , [49] . This work provides a new intellectual framework in which to consider ferroelectric susceptibilities and to explain observations in a range of samples. Our observations provide new insights into the microscopic structural origin of enhanced ferroelectric susceptibilities and a new approach to optimize the properties of epitaxial thin films. Sample preparation 150 nm PbZr 0.2 Ti 0.8 O 3 /10 nm SrRuO 3 or La 0.7 Sr 0.3 MnO 3 /SrTiO 3 (001), (110) and (111) heterostructures were grown via pulsed-laser deposition. The growth of PbZr 0.2 Ti 0.8 O 3 was carried out at an oxygen pressure of 200 mTorr at 635 °C with a laser fluence of 0.9–1.0 J cm −2 and a laser repetition rate of 3 Hz. The growth of SrRuO 3 and La 0.7 Sr 0.3 MnO 3 was accomplished at an oxygen pressure of 100 and 200 mTorr, respectively, at 645 °C with a laser repetition rate of 12 and 3 Hz, respectively. After the growth, the samples were cooled at 5 °C min −1 at an oxygen pressure of 760 mTorr. Crystal and domain structure characterization PFM measurements were carried out using a Cypher AFM (Asylum Research) using Ir/Pt-coated conductive tips (Nanosensor, PPP-NCLPt, force constant~48 N m −1 ). The detailed polarization maps were generated under the single-frequency vector PFM mode that enables the simultaneous imaging of the phase ( θ ) and amplitude ( A ) from both the lateral and vertical piezoresponse signal. To elucidate the PFM contrast, the PFM signals were processed in the form of a combination ( A cos θ ) of phase and amplitude. The X-ray θ –2 θ scans and reciprocal space maps were obtained by high-resolution X-ray diffraction (XPert MRD Pro, equipped with a PIXcel detector, PANalytical). Electrical measurements All the electrical measurements were performed on capacitor structures of PbZr 0.2 Ti 0.8 O 3 films with symmetric electrodes of SrRuO 3 or La 0.7 Sr 0.3 MnO 3 . The patterned circular top electrodes were fabricated by an MgO hard mask technique [50] , and the measurement was conducted on capacitors with the top electrode diameter ranging from 25 to 200 μm. The current–voltage and polarization–electric field hysteresis loops were measured using a Precision Multiferroic Tester (Radiant Technologies, Inc.). The room temperature low-field permittivity and the loss tangent were measured using an E4980A LCR meter (Agilent Technologies). All samples were prepoled prior to the dielectric measurement. During the measurement, the bottom electrode was driven by an AC electric field with an amplitude of 50 mV in the frequency range of 0.1 to 10 kHz. How to cite this article: Xu, R. et al. Stationary domain wall contribution to enhanced ferroelectric susceptibility. Nat. Commun. 5:3120 doi: 10.1038/ncomms4120 (2014).